Social shaping of voices does not impair phenotype matching of kinship in mandrills Kin selection theory provides a strong theoretical framework to explain the evolution of altruism and cooperative behaviour among genetically related individuals. However, the proximate mechanisms underlying kin discrimination, a necessary process to express kin-related behaviour, remain poorly known. In particular, no study has yet unambiguously disentangled mechanisms based on learned familiarity from true phenotype matching in kin discrimination based on vocal signals. Here we show that in addition to genetic background, social accommodation also shapes individual voices in an Old World monkey ( Mandrillus sphinx ), even though primate vocalizations were thought to be innate and little flexible. Nonetheless, social shaping of voice parameters does not impair kin discrimination through phenotype-matching of unknown relatives, revealing unexpected discriminatory versatility despite signal complexity. Accurate signal production and perception, therefore, provide a basis for kin identification and kin-biased behaviour in an Old World primate. Despite ongoing controversies surrounding the importance of kin selection (for example, refs 1 , 2 ), empirical studies have repeatedly demonstrated its major role in determining social relationships in various animal societies [3] , [4] . Whereas kin bias in social behaviour is widespread, the proximate mechanisms underlying the ability to recognize kin remain poorly studied, with the exception of laboratory rodents [5] , [6] . Groups of non-human primates are characterized by the co-residence of individuals belonging to various kin classes and showing variable social bonds [7] . Most groups are also characterized by stable cores of maternally related females (matrilines), enduring mother–offspring bonds and male-biased dispersal [4] , [8] . Learning direct familiarity through social association is certainly the most important mechanism underlying maternal kin discrimination [9] . Because reproduction is often skewed towards one or a few males (for example, ref. 10 ), however, numerous individuals sired by the same father are born into different matrilines. While these paternal kin are less familiar with each other than maternal relatives, they are somehow able to recognize each other as kin because they form stronger social bonds with paternal kin than non-kin [11] , [12] , [13] . Nevertheless, the proximate mechanisms underlying paternal kin discrimination remain poorly known [14] . The phenotype-matching hypothesis explains kin discrimination by holding that an individual matches its own phenotypic traits, or those of known kin, with those of unknown individuals to assess kinship [5] , [15] . Testing this mechanism unambiguously is challenging because pairs of individual subjects should never have interacted socially before the experiment, so as to exclude the confounding process of learning direct familiarity [14] . Here we take advantage of a unique setting in three Gabonese populations of mandrills, a typical matrilineal primate society with high male reproductive skew [16] , to study the potential role of contact calls in kin discrimination and kin-biased behaviour. These populations have been extensively studied for the past 10–30 years (for example, refs 17 , 18 ), and their complete pedigrees are available. Moreover, these populations are historically linked, and a subset of related individuals never met. This situation enabled us (i) to investigate the joint effect of relatedness and familiarity on features of calls and (ii) to perform a conclusive test of the phenotype-matching hypothesis, using vocalizations as signals. In particular, using a combination of acoustic analyses and playback experiments, we demonstrate that mandrill’s vocalizations contain kin-specific information and that individuals actually use this information. This study distinguishes the mechanisms of learning direct familiarity from true phenotype-matching in kin-discrimination processes based on vocal cues. However, we also demonstrate that mandrill vocalizations are modulated by their social environment. This second result is important regarding recurrent discussions about genetically determined versus socially influenced, or learned, call structure in non-human primates. Their vocalizations are still thought to be largely innate with little flexibility in call structure or usage (but see refs 19 , 20 , 21 , 22 , 23 ). 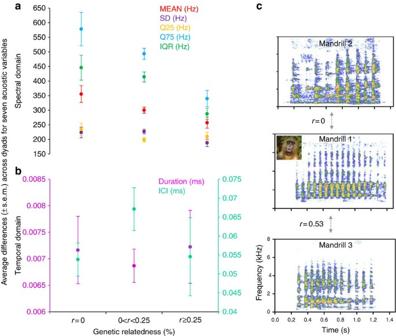Figure 1: Acoustic differences across dyads as a function of their genetic relatedness for seven variables. The seven variables belong to (a) the spectral domain (mean frequency ‘MEAN’ in red, s.d. of the mean frequency SD in purple, first quartile ‘Q25’ in orange, third quartile ‘Q75’ in blue, interquartile range ‘IQR’ in green) and (b) the temporal domain (call ‘DURATION’ in pink, intercall interval ‘ICI’ in light green). For the sake of clarity, we represent average acoustic differences (±s.e.m.) as a function of three levels of relatedness. The three spectrograms (c) on the right of the figure illustrate the acoustic similarity between calls according to relatedness: mandrills 1 and 2 are unrelated (r=0); mandrills 1 and 3 are related (r=0.53). Familiarity and genetic ties impact mandrill vocalizations We show that the acoustic structure of contact calls recorded from 36 male and female mandrills ( Supplementary Table 1 ) with different levels of relatedness and familiarity ( Supplementary Tables 2 and 3 ) is more similar among relatives than among unrelated individuals, when controlling for other confounding effects (see Methods), including familiarity (calculated as the number of years spent in the same social group). Indeed, of the seven acoustic variables examined to characterize the vocal signature of individuals, genetic relatedness alone or genetic relatedness in interaction with familiarity influence four out of five variables belonging to the spectral domain and one out of two variables belonging to the temporal domain (General Linear Mixed Model—LMM; Table 1 and Fig. 1 ; see Methods). Moreover, the resulting acoustic distance across dyads in the space defined by the first two principal component analysis (PCA) components calculated from the seven orthogonally transformed acoustic variables (Euclidean acoustic distances) is also significantly influenced by relatedness in combination with familiarity (LMM, N =630 dyads, F 1,628 =7.87, P =0.0052; Table 1 ). Acoustic distance decreases with familiarity but this decrease is more pronounced when relatedness is low ( Supplementary Fig. 1 ). In particular, among unfamiliar dyads—the ones that have never experienced any form of social contact—the highly related dyads are the ones that are acoustically the most similar ( Fig. 2a ). Our results further indicate that familiarity and relatedness tend to have an impact on acoustic parameters in different ways ( Table 1 ). Although it is unlikely that any of the acoustic variables is entirely innate or learned, some acoustic variables might be more influenced by relatedness (‘innate’ features) and thus should be less flexible than those more influenced by familiarity (‘learned’ features). For instance, a variable representing the fluctuation of the mean frequency (that is, SD frequency) should be more plastic than the mean frequency itself. Our results are in line with this reasoning where the SD frequency is significantly influenced by familiarity, while mean frequency of the call spectrum (MEAN) frequency is more sensitive to relatedness ( Table 1 ). Table 1 Predictors of seven acoustic variables. Full size table Figure 1: Acoustic differences across dyads as a function of their genetic relatedness for seven variables. The seven variables belong to ( a ) the spectral domain (mean frequency ‘MEAN’ in red, s.d. of the mean frequency SD in purple, first quartile ‘Q25’ in orange, third quartile ‘Q75’ in blue, interquartile range ‘IQR’ in green) and ( b ) the temporal domain (call ‘DURATION’ in pink, intercall interval ‘ICI’ in light green). For the sake of clarity, we represent average acoustic differences (±s.e.m.) as a function of three levels of relatedness. The three spectrograms ( c ) on the right of the figure illustrate the acoustic similarity between calls according to relatedness: mandrills 1 and 2 are unrelated ( r =0); mandrills 1 and 3 are related ( r =0.53). 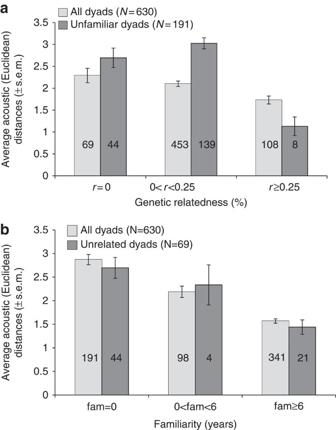Figure 2: Acoustic distances and genetic relatedness and familiarity. The average acoustic distances across all dyads (light grey) and across all unfamiliar dyads (a) or across all unrelated dyads (b; dark grey) as a function of their genetic relatedness or familiarity (respectively) are shown. Euclidean acoustic distances were calculated from seven acoustic variables that were represented in a two-dimensional PCA space. For the sake of clarity, we represent average acoustic distances (±s.e.m.) as a function of three levels of relatedness or three levels of familiarity (in years). Numbers within bars give the sample sizes for each level. Full size image Figure 2: Acoustic distances and genetic relatedness and familiarity. The average acoustic distances across all dyads (light grey) and across all unfamiliar dyads ( a ) or across all unrelated dyads ( b ; dark grey) as a function of their genetic relatedness or familiarity (respectively) are shown. Euclidean acoustic distances were calculated from seven acoustic variables that were represented in a two-dimensional PCA space. For the sake of clarity, we represent average acoustic distances (±s.e.m.) as a function of three levels of relatedness or three levels of familiarity (in years). Numbers within bars give the sample sizes for each level. Full size image Restricting the data set to dyads that are strictly unfamiliar, the degree of relatedness remains the only predictor influencing acoustic distances (LMM, N =191 dyads, F 1,189 =9.42, P =0.0026; Log-likelihood Ratio Test (LRT)—comparing full versus null models: D =19.3, P <0.01; Fig. 2a ). Similarly, restricting the analyses to unrelated dyads, we found that more familiar dyads exhibit more similarity in their acoustic features than more unfamiliar dyads (LMM, N =69 dyads, F 1,67 =11.33, P =0.002; LRT: D =18.4, P <0.01; Fig. 2b ). Finally, the study of the effect of kin classes, considering maternal half-siblings, paternal half-siblings and non-kin dyads alone ( N =100 dyads), revealed a significant effect of kinship in combination with the degree of familiarity of the dyad: maternal and paternal half-siblings are acoustically more similar than non-kin dyads, especially when they are unfamiliar or little familiar with each other (LMM, N =100 dyads, F 3,95 =4.86, P =0.013; Table 2a ; Fig. 3 ). Interestingly, maternal half-siblings tend to be acoustically more similar than paternal half-siblings ( Table 2b ; Fig. 3 ), despite similar relatedness coefficients ( r ∼ 0.25). Table 2 Kinship and acoustic distance. 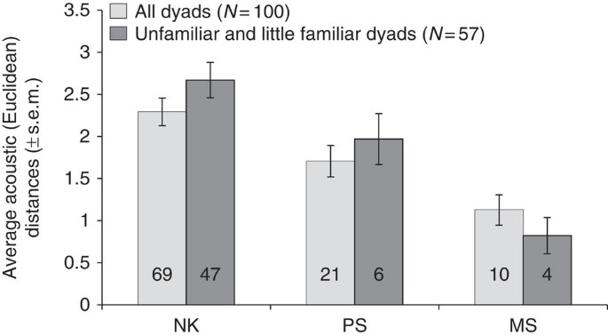Figure 3: Acoustic distances and kinship and familiarity. The average Euclidean acoustic distances across all dyads (light grey) and across all unfamiliar or little familiar dyads (individuals that lived less than 3 years together; dark grey) as a function of three kin classes (maternal half-siblings, MS; paternal half-siblings, PS; non-kin, NK) are shown. Euclidean acoustic distances (±s.e.m.) were calculated from seven acoustic variables that were represented in a two-dimensional PCA space. Sample sizes for each relatedness level are given (numbers within bars). Full size table Figure 3: Acoustic distances and kinship and familiarity. The average Euclidean acoustic distances across all dyads (light grey) and across all unfamiliar or little familiar dyads (individuals that lived less than 3 years together; dark grey) as a function of three kin classes (maternal half-siblings, MS; paternal half-siblings, PS; non-kin, NK) are shown. Euclidean acoustic distances (±s.e.m.) were calculated from seven acoustic variables that were represented in a two-dimensional PCA space. Sample sizes for each relatedness level are given (numbers within bars). Full size image Taken altogether, these results indicate that mandrill vocal signals convey reliable information on genetic relatedness and that social accommodation further modifies individual voices. Indeed, the degree of familiarity influences individual acoustic features, and unrelated but familiar individuals exhibit voice similarities. In addition, maternal half-siblings appear to be the most acoustically similar kin (albeit only showing a nonsignificant trend in this direction in comparison with paternal half-siblings). These maternal kin live in a more close-knit social environment than do paternal half-siblings. Social environment (familiarity) and probably social ties (maternal kinship) may therefore modulate voice features, as does genetic information. Whereas vocal plasticity at the individual level is well documented in songbirds [24] , parrots, dolphins and seals [20] , studies showing socially guided flexibility in primate calls are still sparse (for example, refs 25 , 26 , 27 ). Conversely, several studies have shown the vocal repertoire of primates to be fixed and genetically determined. For example, social isolation or early deafness does not prevent squirrel monkeys from spontaneously producing the full vocal repertoire of their species [28] . Cross-fostered macaques raised with individuals from a different species still continue to produce their own species-specific calls [29] . Genetic factors therefore seem to determine the general species-specific vocal repertoire of a primate species; however, social factors can modify some calls, which may then function as a ‘social badge’ [22] in the same way as described for humans [30] . True phenotype matching in mandrills is based on vocal cues Using playback experiments, we tested the phenotype-matching hypothesis by studying 101 sender–receiver dyads with different levels of relatedness and familiarity ( Supplementary Table 3 ). We found that receivers respond more intensely (more body and head movements towards the speaker, including travelling movements) to the calls of related senders (Generalized Linear Mixed Model—GLMM; controlling for other factors: F 1,99 =7.12, P =0.010; Table 3 and see Methods). In contrast, the degree of familiarity between senders and receivers does not influence receivers’ responses ( F 1,99 =0.83, P =0.37). When we restricted our analysis to strictly unfamiliar sender–receiver dyads ( Supplementary Table 3 ), genetic relatedness is the strongest predictor influencing receivers’ responses: there are twice as many behavioural responses induced by calls from related individuals ( r ≥0.25) than from unrelated individuals (GLMM; N =59, F 1,57 =3.67, P =0.073; Fig. 4 ), although this effect only approaches significance owing to low sample size. Table 3 Predictors of playback responses. 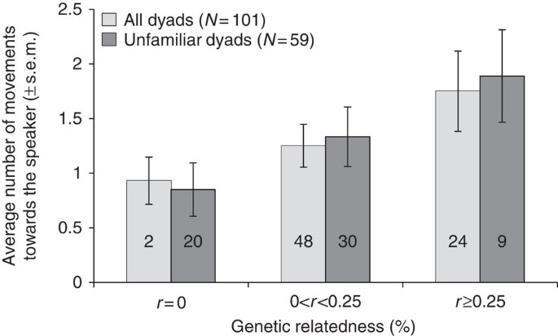Figure 4: Playback responses and genetic relatedness. The playback responses (average number of movements displayed towards the speaker±s.e.m.) as a function of sender–receiver’s genetic relatedness, across all dyads (light grey) and across unfamiliar dyads only (dark grey) are shown. For the sake of clarity, three classes of genetic relatedness are represented. Sample sizes for each relatedness level are given (numbers within bars). Full size table Figure 4: Playback responses and genetic relatedness. The playback responses (average number of movements displayed towards the speaker±s.e.m.) as a function of sender–receiver’s genetic relatedness, across all dyads (light grey) and across unfamiliar dyads only (dark grey) are shown. For the sake of clarity, three classes of genetic relatedness are represented. Sample sizes for each relatedness level are given (numbers within bars). Full size image Evidence for the importance of acoustic kin discrimination has also recently been found in two other primate species. Captive female-grey mouse lemurs ( Microcebus murinus ) responded differently to calls from their fathers compared with unrelated males [31] , and female rhesus macaques ( Macaca mulatta ) responded more often to calls from unfamiliar paternal half-sisters than to those from unrelated females [32] . However, female lemurs and their fathers were kept together as adults for variable periods of time so that caller identity could have been linked to other cues of relatedness. Moreover, the unfamiliar pairs in the macaque study, although from different social groups, lived on the same small island where intergroup encounters are frequent. Direct familiarity among subjects can therefore also not be completely excluded. Our study, therefore, unravels a proximate mechanism that plays a significant role in kin-discrimination processes, demonstrating unequivocal support for the phenotype-matching hypothesis through vocal signals. In summary, our study reveals that primate vocalizations can be shaped by both genetic factors and social experience. Mandrills’ contact calls contain information about genetic relatedness and the degree of familiarity between individuals. Mandrills are also able to rely on these complex vocal signals alone to discriminate unknown kin from non-kin. Accurate signal production and perception therefore provide a basis for kin identification and kin-biased behaviour. Because mechanisms of phenotype matching rely on communication systems that include the emission of signals, their transmission throughout the environment and their reception and processing by receivers [33] , imperfect coding or decoding may occur all along this chain. Other communication channels might, therefore, be involved simultaneously to reinforce the signal. Mandrills live in large groups comprising several hundred individuals, and both visual and olfactory signals may signal relatedness at short distances. In contrast, in closed forest habitats, vocal signals may enable individuals to adjust their behavioural responses to more distant senders. The present study on acoustic kin discrimination in an Old World primate therefore reveals an unexpected discriminatory versatility despite previously unknown signal complexity. Population information We studied three mandrill populations living in southern Gabon. A semi-free ranging population (hereafter termed ‘semi-free population’) composed of ∼ 200 individuals lives in two contiguous forested enclosures (9.5 ha) at the Centre International de Recherches Médicales de Franceville (CIRMF). CIRMF also houses a captive population (hereafter termed ‘caged population’) composed of 13 individuals (10 individuals originated from the semi-free ranging population and three were wild-caught animals). The caged population is located ∼ 1 km away from the semi-free population so that the two populations do not experience acoustic contact. The captive individuals are socially housed in three neighbour cages (6.5 m × 7.5 m × 2.5 m) with permanent audio, visual and potential physical contact among them. Each of the three subgroups was composed of two to four adult females and one to two adult males. Both the caged and the semi-free populations originated from 14 wild unrelated founders that arrived at CIRMF in the early 1980s (for example, refs 11 , 34 ). Caged and semi-free animals are related to different degrees; however, some kin never experienced any social contact with each other since animals from both populations continued to reproduce throughout the years. Finally, a wild population (hereafter termed ‘wild population’) composed of ∼ 120 individuals lives in a private park in southern Gabon (Parc de la Lékédi, Bakoumba). About 20% of the individuals from this population originated from the semi-free population from CIRMF, released in 2002 and 2006. From 2002 on, wild adult and sub-adult males immigrated into this group and sired offspring with the released females and their descendants [18] . Again, the two CIRMF populations and the wild population contain individuals that are genetically related to various degrees but that never met. For this study, we recorded calls from a total of 39 individuals belonging to the semi-free ranging ( N =34) and the wild ( N =5) populations (a subset of 36 individuals were used for the acoustic analyses including the five wild animals; see below), and we performed playback tests on 13 captive receivers ( Supplementary Table 2 ). Individuals in all three populations are habituated to humans and are individually recognized as a result of daily population monitoring. Behavioural follows-ups allowed us to determine the exact age of all study individuals and to assign a dominance rank, unambiguously attributed following methods based on approach-avoidance behaviour [35] . In all subsequent analyses, we considered three classes of dominance rank (high-, mid- and low-ranking animals). All individuals of the three mandrill populations are regularly captured using blowpipe intramuscular injections of anaesthetics (for example, refs 16 , 36 ), and blood samples are collected on every occasion. DNA extractions from white cells were performed using QIAamp DNA Blood Mini Kits (Hilden, Germany) and microsatellite genotyping was carried out using 12 primer pairs (as per ref. 16 ). Paternity analyses were performed using Cervus 3.0 software using previously described procedures [16] . We were able to reconstruct the full pedigree of all study individuals, going back as far as the generation of the founder animals that were all unrelated (four to five maternal generations in total). We also reconstructed the full pedigree of each of the five sampled wild animals, all of which originated from the semi-free ranging population. For each dyad (sender–sender for the acoustic analysis and sender–receiver for the playback analysis), we were therefore able to assign an exact coefficient of genetic relatedness. For example, mother–offspring dyads were related at 0.5. However, most studied dyads were related through both the paternal and the maternal lines (of ‘mixed origin’ as in Supplementary Table 3 ) because of limited male migration and subsequent inbreeding. For the acoustic analyses alone, sample sizes allowed distinguishing dyads of true non-kin from paternal and maternal half-siblings. In these analyses, paternal half-siblings did not come from the same matriline and maternal half-siblings did not share a common father. By contrast, in the playback analyses, limited sample sizes did not allow examining differences among kin classes. In all our analyses, we were also able to control for the degree of familiarity between individuals. Two individuals were considered as familiar when they experienced any form of social contact during a stage of their life. Familiar individuals spent between 6 months to almost 23 years together (there were no familiar dyads that lived for less than 6 months together in the studied population; mean±s.d. across all studied dyads: 4.5±4.3 years). In the following analyses, we considered the number of years living in the same social environment rounded to the higher nearest integer as a conservative estimate of familiarity. However, because some of the dyads were familiar to each other several years ago (then subsequently separated), while others were familiar only a few years ago or are still familiar, we re-ran all analyses using ancient versus recent familiarity as an explanatory variable. The age of familiarity had an impact on neither the studied acoustic parameters nor the playback responses ( Supplementary Note 1 ). This study complies with ethical protocols approved by the CENAREST institution (authorization number: AR0003/12/MENESRSIC/CENAREST/CG/CST/CSAR). The research adhered to the legal requirements of Gabon for the ethical treatment of non-human primates. Acoustic analyses In April 2013, we recorded contact calls (‘kakak’) of 36 males and females ( Supplementary Tables 1 and 2 ). These calls are naturally produced by females of any age and non-adult males when the group starts to move, and more generally when individuals need to know where conspecifics are (see also ref. 37 ). These calls are composed of typical sequences of several consecutive calls (on average eight calls per sequence, range 2–21, N =84 sequences; Fig. 1 and Supplementary Audio Files 1–3 ). Mandrill contact calls have a wide frequency spectrum with a harmonic structure that is more or less visible ( Fig. 1 ). They are short in duration (mean±s.d. : 33±9 ms) and can be modulated in frequency and amplitude ( Supplementary Table 1 ). Contact calls were recorded with a Sennheiser MKH70 ultra directional microphone connected to an H4n ZOOM digital recorder (resolution: 16 bits; sampling rate: 44.1 kHz; Waveform Audio File format). Recordings were performed during direct observations of mandrills foraging in clear forest understory for the wild population and around feeding time from an observation platform for the semi-free population. Recordings were all performed between 5 and 10 m from the sender, with no obstacle between the sender and the microphone. The identity of each sender was immediately double-checked with at least one additional observer. We extracted temporal and spectral parameters from 526 calls of 84 sequences of contact calls displayed by 36 individuals (mean±s.d. : 14.6±10.3 calls per individual, range: 3–41; 2.4±1.4 sequences per individual, range: 1–6). The individuals for which we obtained a small number of calls were not more or less related to other study animals than expected by chance and were therefore unlikely to have biased our results. Calls were analysed with a dedicated R script built from the package ‘Seewave’ version 1.6.7 (ref. 38 ), especially committed to sound processing. We carefully checked each call by visualizing its spectrogram using the Praat version 5.3.56 DSP package devised by P. Boersma and D. Weenink (University of Amsterdam, the Netherlands, www.praat.org ) to ensure the absence of any transient background noise (bird, cicada, other mandrills). When necessary, we manually corrected the onset and/or the offset of calls to be targeted by the script and discarded the measurements of calls that were overlapped by a background sound. We ran the script in the frequency bandwidth between 120 and 5,000 Hz. Overall, our script measured seven acoustic variables from each analysed call. These variables describe the acoustic structure in both the temporal and the spectral domains and are commonly used to assess vocal signatures embedded in sound signals [39] , [40] . Two variables belonged to the temporal domain (in ms): the total duration of calls (hereafter DURATION) and the silence duration (intercall interval; ICI) between the offset of the previous call and the onset of the considered call. Three spectral variables described the distribution of energy over the duration of the call (in Hz): the frequency value at the upper limit of the first quartile of energy (Q25), the frequency value at the upper limit of the third quartile of energy (Q75) and the interquartile range (IQR). Last, we considered two additional spectral parameters (in Hz): the mean frequency of the call spectrum (MEAN) and the standard deviation of the mean frequency (SD). For each of these seven acoustic variables, we performed statistical analyses taking into account the absolute differences between all dyads of individuals involving 36 senders ( N =630 dyads). To obtain acoustic measures in two dimensions for each call, we performed a PCA on scaled variables with Statistica 6 software (Statsoft Inc., 2001). We considered the two first factors of the PCA (representing 68.6% of the total variance) as call coordinates. The first component was mainly explained by Q75 (28.6%) and MEAN (25.5%), and the second component by Q25 (46.6%). For each individual, we then calculated an average acoustic measure (or barycenter) from the call coordinates. Last, we calculated the Euclidean acoustic distance between all dyads of individuals based on the individual coordinates. To sum up, for each dyad, we obtained eight values: one average absolute difference for each of the seven acoustic variables and one Euclidean acoustic distance. To study the effect of genetic relatedness (ranging from 0 to 0.69 among the study subjects) and familiarity (ranging from 0 to 23 years) on these acoustic features, we first performed General Linear Mixed Models (LMM, Proc GLIMMIX, SAS v9.4) with a Gaussian error structure. Normality of the residuals was attained after applying the following transformations: Euclidean acoustic distance, MEAN, Q25, Q75, IQR and DURATION were square root-transformed; ICI was ln-transformed; SD was kept untransformed. We further considered the following predictors as possible confounding covariates: whether the two individuals of the dyads belonged to the same population or not (discrete variable coded 0 or 1), the sex composition of the dyad (discrete variable coded female-female, male-female or male-male), the difference in age (absolute age difference between members of a dyad) and the absolute difference in dominance rank (continuous variable ranging from 0 to 2, see above). We also considered the identity of the two senders as two random effects. Second, we performed two more LMM based on the acoustic distance, restricting our data first to the strictly unfamiliar dyads and then to the strictly unrelated dyads. In a final analysis, we further explored the effect of kinship on the acoustic distance for a subset of dyads including non-kin, paternal half-siblings and maternal half-siblings, as described above. We compared these three classes of kin using differences in least-square means (lsmeans procedure, SAS v9.4). Whenever necessary, we applied Holm–Bonferroni corrections for multiple testing (see Table 1 ). For these LMM, we also verified that full models with all predictors produced significantly better fit than null models (that is, models considering the intercept and random effects only), using LRT [41] . Finally, we checked for the absence of co-linearities and multicolinearities among the predictors using variance of inflation criteria (Proc REG, SAS V9.4; variance of inflation<2 in all instances). We also checked for the stability of the models by randomly excluding some data points. Playback experiments We selected contact calls of 19 adult females ( N =23 sequences; Supplementary Table 4 ) according to their relatedness and familiarity with the ‘receivers’ ( Supplementary Tables 2 and 3 ). The call sequences lasted on average 984±184 ms and included 9.6±3.6 calls, each call were spaced on average by 71.9±41.1 ms of silence. The MEAN frequency of the calls was 1,774±284 Hz. The sequences were played twice with an interval of 8 s. This coding strategy based on the redundancy of signals aims to increase the receiver’s attention (see for review ref. 42 ). The sequences were prepared using the GoldWave software v5.68 and their intensity was normalized. All receivers ( N =13; Supplementary Table 2 ) belonged to the caged population and were tested in their usual social environment (see above) to not disturb or stress the animals by temporarily isolating them. At the beginning of the playbacks, all studied receivers were already habituated to our presence and to the devices used, and did not show any visible signs of disturbance. Because the receivers were not acoustically isolated from each other, we carefully scheduled the playback experiments to test the different types of relationships while limiting the number of playback sessions to avoid habituation. In total, we performed 36 playback sessions and examined the behavioural responses of 101 sender–receiver dyads. Sender–receiver relatedness and familiarity were exactly known for each dyad. To optimize the number of playback sessions, three to four observers, who were blind regarding the relatedness and the familiarity of sender–receiver dyads, stood around the cages at ∼ 1.5 m from the fences to monitor all focal receivers, which were randomly assigned. Each observer monitored several times each receiver with different combination of sender–receiver characteristics of familiarity and relatedness. Using vocal recorders, we thus recorded simultaneously the responses of three to four receivers. All behavioural responses were then coded by one person who was also blind regarding the relatedness and the familiarity of sender–receiver dyads. For each session, the positions of the observers, the microphone (Sennheiser MKH70 ultra directional microphone) on a tripod and the loudspeaker connected to a laptop were changed to avoid habituation. The loudspeaker was hidden in the vegetation at the edge of the forest in four random locations surrounding the cages (8–12 m away). Call sequences were played back at natural amplitude (73±1 dB SPL measured at 1 m with a Bioblock Scientific sound level meter). They were broadcast using an amplified portable speaker Premio 8 (70 W, frequency response: 70 Hz to 20 kHz). Sounds were played back when the receivers were not involved in social interactions. Examination of the playback data revealed that the response of each receiver was independent of the responses of the other tested receivers. To avoid associations between the presence of observers and the broadcast sound, we performed ‘mock sessions’ during which the observers were equipped with recording equipment and stood by the cages recording behavioural data on focal individuals. The full equipment was set up to imitate the conditions of real playback sessions. Three days before starting the first playback session, we performed these ‘mock sessions’ twice a day, every day. We then randomly performed ‘mock sessions’ throughout the period of the experiment. Over a month, four sessions of 30 min each were performed every day. Two sessions occurred at noon and two sessions at 16:00 h (after feeding). Two consecutive sessions were separated by a pause of 20 min. The number and the order of playback sessions were randomized from none (only ‘mock sessions’ occurred) to three sessions per day (along with one ‘mock session’). If a same sequence of calls had to be broadcast more than once, the two sessions were performed at least 2 days apart. Most of the sequences were used once (60.9% of the sequences), the others were played twice (30.4%). Only one sequence (4.3%) was played three or five times, respectively. To assess the intensity of the response of receivers, we recorded any changes in their behavioural activities during the minute following the stimulus, a time period that allowed the receivers to return to their baseline activity. Changes of activity included travelling and changes in postures such as body and head movements (for example, turning the head, getting up, sitting down, moving and putting the arms on the fence) and their direction (towards the loudspeaker or any other direction). To investigate the factors explaining the intensity of the receivers’ responses (total number of body and head movements in the direction of the loudspeaker), we ran a Generalized Linear Mixed Model (GLMM, Proc Glimmix, SAS v9.4) with a negative binomial distribution and logit link-function for count data because data were slightly overdispersed compared with expectations under a Poisson distribution (variance>mean). We included as fixed effects the relatedness coefficient between the sender and the receiver (ranging from 0 to 0.5) and their degree of familiarity (number of years spent in the same social environment, ranging from 0 to 11 years). We further considered several characteristics of the receiver including sex (male/female), age and dominance rank ( Supplementary Table 2 ). Dominance rank was considered as a discrete variable where a male’s rank was either 1 (dominant) or 2 (subordinate) because there were never more than two males in one social group, and where a female’s rank ranged from 1 (dominant) to 3 (subordinate). In addition, we considered senders’ characteristics including population identity (discrete variable coded 0 or 1), as well as age and dominance rank (all senders were females). Dominance rank of senders was a discrete variable ranging from 1 to 3 as described above ( Supplementary Table 2 ). We further included the number of times that a given sequence of calls from a similar sender was broadcast over the 30-day experimental period (continuous variable ranging from one to five times, see above). This variable was highly correlated with the cumulative number of times each receiver was previously exposed to playbacks (namely the number of playback sessions already broadcast), therefore mimicking habituation effects. This cumulative number of times animals were exposed to playbacks showed the same effect as the number of emissions of the same sequence of calls and did not change our results concerning relatedness ( Supplementary Note 2 ). We chose to keep the number of emissions of a same sequence of calls in our analysis as a fixed effect. We also considered the number of body and head movements displayed towards any direction other than the loudspeaker to correct for the possible hyperactivity of some receivers. Finally, we considered the identity of the receivers ( N =13), the identity of the senders ( N =19) and identity of the playback sessions ( N =36) as three random effects. Over 19 senders, only four individuals had two different sequences of call broadcast, precluding the use of an additional random effect of call sequence identity. We, however, performed two additional analyses. First, we re-ran the playback analysis using the call sequence identity as a random effect rather than the sender identity. Second, we restricted our data set to a single call per individual (chosen randomly) leading to a situation free of pseudoreplication. In both cases, results did not change qualitatively ( Supplementary Note 3 ). As above, we verified that full models produced significantly better fits than null models using LRT. We also checked for the absence of co-linearities and multicolinearities among the predictors (variance of inflation<2 for all predictors). We further verified the stability of the models by randomly excluding some data points. Finally, for this playback analysis, we did not replace genetic relatedness by the kin classes of the studied dyads because of numerous mixed (paternal and maternal) ancestries. We instead re-ran our model considering only the non-familiar dyads that never met once in their life. How to cite this article: Levréro, F. et al. Social shaping of voices does not impair phenotype matching of kinship in mandrills. Nat. Commun. 6:7609 doi: 10.1038/ncomms8609 (2015).